Soil clay content underlies prion infection odds Environmental factors—especially soil properties—have been suggested as potentially important in the transmission of infectious prion diseases. Because binding to montmorillonite (an aluminosilicate clay mineral) or clay-enriched soils had been shown to enhance experimental prion transmissibility, we hypothesized that prion transmission among mule deer might also be enhanced in ranges with relatively high soil clay content. In this study, we report apparent influences of soil clay content on the odds of prion infection in free-ranging deer. Analysis of data from prion-infected deer herds in northern Colorado, USA, revealed that a 1% increase in the clay-sized particle content in soils within the approximate home range of an individual deer increased its odds of infection by up to 8.9%. Our findings suggest that soil clay content and related environmental properties deserve greater attention in assessing risks of prion disease outbreaks and prospects for their control in both natural and production settings. For over two centuries, environmental factors—especially soil properties—have been suggested as being potentially important in the epidemiology of scrapie [1] , [2] , [3] , [4] , the infectious prion disease of sheep and goats. Moreover, some reservoir of infection or infectivity has long been suspected for scrapie [1] , [2] , [3] , [4] , [5] , [6] , [7] , [8] and also for chronic wasting disease [9] , [10] , [11] , a strikingly similar prion disease of species in the deer family. Scrapie and chronic wasting disease prions can be transmitted from animal and environmental sources [3] , [5] , [8] , [12] , [13] , [14] , [15] . Although infected animals most likely carry prions between locations, environmental conditions may affect if transmission and outbreaks follow once prions have been introduced. Soil characteristics could be a source of environmental influence on prion epidemic dynamics by affecting host susceptibility [16] , [17] , [18] or by modulating prion infectivity or persistence [16] , [19] , [20] , [21] , [22] , [23] , [24] , [25] , [26] . Soil itself has been suggested as a logical medium for harbouring prions [3] , [4] , [5] , [12] , [14] , [19] , [20] , [25] , [26] . Some phyllosilicate clay minerals (for example, montmorillonite and kaolinite) [19] , [20] , [26] , quartz microparticles [19] , [26] , [27] and soils enriched with these particles [20] , [25] , [26] can bind to prions and enhance both their persistence and their infectivity, thereby offering a plausible mechanism for such harbouring. In addition to phyllosilicate and quartz microparticles, organic polyanions [21] , manganese [23] , [24] and other soil components [20] , [22] also have some capacity for interaction with prions in simulated conditions and thus could influence bioavailability and persistence of prions in the environment. Because both montmorillonite microparticles and phyllosilicate-bearing soils had been shown to facilitate prion transmission experimentally [19] , [20] , we hypothesized that prion transmission among mule deer ( Odocoileus hemionus ) might be enhanced in individual home ranges with locally high soil clay content (that is, a large proportion of the soil particles are <2 μm in size). In this study, we report apparent effects of soil clay particle content on the odds of prion infection in individual mule deer. Our application of Bayesian hierarchical spatial models to georeferenced data from prion-infected deer populations and local landscape features revealed that increasing mean soil 'clay' content (expressed as the percentage of soil particles sized <2 μm) within the 9 km 2 area approximating the home range of an individual mule deer [28] , [29] ('vicinity' hereafter) was associated with increased odds of prion infection in both northcentral and northwestern Colorado, USA. Our findings suggest that soil clay content and related environmental properties deserve greater attention in assessing risks of prion disease outbreaks and prospects for their control. Northcentral Colorado study area The effect of soil clay content on the odds of infection was most evident in northcentral Colorado ( Fig. 1a ) where prion disease has occurred since at least from the 1960s (ref. 9 , 30 ). In this area, the average soil clay content in the vicinity of sampled deer ranged from 4 to 32% and the odds of prion infection increased by 8.9% for every 1% increase in soil clay (odds ratio 1.089; 95% credible interval (CI) 1.038–1.141). 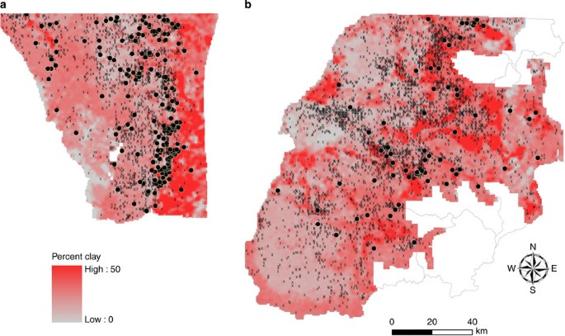Figure 1: Spatial relationships between soil clay content and prion disease in mule deer. (a) The average percentage of clay-sized particles contained in soils37,48within the 9 km2area surrounding a sampled deer strongly influenced its odds of prion infection in northcentral Colorado, USA (Table 1). (b) A similar relationship between soil clay content and the odds of prion infection also was evident in deer sampled from northwestern Colorado (Table 1). In both panels, dots (•) represent locations of prion-infected deer presence and crosses (×) represent locations of apparently uninfected deer presence. Percent clay within the vicinity of sampled deer was by far the most important variable in the best model to explain infection probability ( Table 1 ). Moreover, percent clay was included in the top four models to explain infection probability ( Supplementary Table S1 ). These four models clearly represented the best fitting of those considered ( Supplementary Table S1 , 'Weights'), providing strong evidence that including the percent clay parameter enhanced these models' abilities to explain the underlying infection-generating process far better than similar models in the candidate set lacking the parameter [29] , [31] , [32] . Figure 1: Spatial relationships between soil clay content and prion disease in mule deer. ( a ) The average percentage of clay-sized particles contained in soils [37] , [48] within the 9 km 2 area surrounding a sampled deer strongly influenced its odds of prion infection in northcentral Colorado, USA ( Table 1 ). ( b ) A similar relationship between soil clay content and the odds of prion infection also was evident in deer sampled from northwestern Colorado ( Table 1 ). In both panels, dots (•) represent locations of prion-infected deer presence and crosses (×) represent locations of apparently uninfected deer presence. Full size image Table 1 ∣ Parameter estimates from best-fitting models. Full size table Northwestern Colorado study area In northwestern Colorado ( Fig. 1b ), where prion disease was introduced more recently and infection rates are relatively low, percent clay in soil in the vicinity of sampled deer ranged from 0 to 38%. There, the odds of prion infection increased by 3.9% for every 1% increase in local soil clay (odds ratio 1.039; 95% CI 1.002–1.079). Similar to our findings in the northcentral area, percent clay within the vicinity of deer sampled in the northwest was the most important variable in the best model to explain infection probability ( Table 1 ) and was included in two of the three best explanatory models ( Supplementary Table S2 ). Other influences on prion infection odds Our analyses, which simultaneously adjusted for other covariates and spatial structure in the data, reaffirmed that a mule deer's age, sex and other habitat features within its likely home range also influence its odds of prion infection ( Table 1 , Supplementary Tables S1−S2 ). Our findings support the notion that soil may have an important role in perpetuating epidemics of infectious prion diseases [1] , [2] , [3] , [4] , [5] , [11] , [12] , [16] , [19] , [20] , [25] , [26] , perhaps by serving as an environmental reservoir for prions. Other soil attributes may modulate prion bioavailability and infectivity in natural environments [16] , [19] , [20] , [21] , [22] , [23] , [24] , [25] , [26] , [27] , but soil clay content alone seems to offer a parsimonious improvement towards explaining spatial patterns of prion infection among mule deer inhabiting montane ranges of northern Colorado. Some chronic wasting disease foci in Colorado and elsewhere in western north America [33] overlap areas where surface soils have a relatively high cation exchange capacity [34] ( Fig. 2 ). Such soils tend to have high clay content and/or high organic matter content [35] . The soils in our two study areas contain high proportions of phyllosilicate and quartz microparticles [36] and relatively little organic matter [37] and thus appear very similar in composition to other soils shown to enhance prion persistence [25] or oral transmissibility [20] . Because soils with relatively high clay content relative to organic matter (for example, clay/organic matter ratio >1:1) may have a greater tendency to enhance prion transmission [20] , a ratio of percent clay to percent organic matter also might be useful for assessing landscape-level associations between soil characteristics and potential prion transmission risk in areas with higher organic matter content than encountered in our study areas. 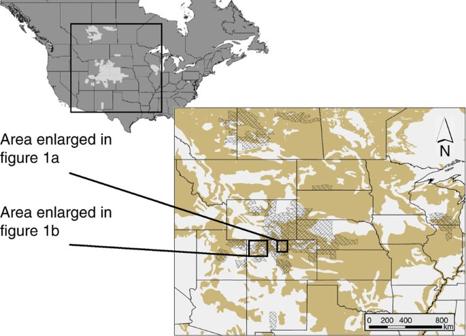Figure 2: North American distribution of prion disease in deer. In some areas, prion disease foci in deer (Odocoileusspp.) in western North America33overlap landscapes with soils that have cation exchange capacity (CEC)34values (tan areas in inset) suggestive of a relative abundance of clay minerals (phyllosilicates) and/or organic matter. Game management units (GMUs) are administrative boundaries used in hunting management30,47; prion-infected GMUs are shown in light grey on the continental map and in cross hatching on the inset. Figure 2: North American distribution of prion disease in deer. In some areas, prion disease foci in deer ( Odocoileus spp.) in western North America [33] overlap landscapes with soils that have cation exchange capacity (CEC) [34] values (tan areas in inset) suggestive of a relative abundance of clay minerals (phyllosilicates) and/or organic matter. Game management units (GMUs) are administrative boundaries used in hunting management [30] , [47] ; prion-infected GMUs are shown in light grey on the continental map and in cross hatching on the inset. Full size image Although the fine-scale soil data available for analysis here did not include mineralogical composition estimates, we believe that percent clay was a meaningful index for (if not a direct measure of) the relative abundance of clay minerals shown experimentally to enhance oral prion transmission [19] , [20] , [26] . The clay-bearing soils in our study areas were derived from Cretaceous shales (Pierre shale in the northcentral area, Mancos shale in the northwest) [38] , [39] , with high smectite content [36] , [38] , [40] . The clay-sized particle fractions of representative surface soils arising from these shales contain high proportions of montmorillonite (26−40%), kaolinite (10−11%) and quartz microparticles (8−10%)(ref. 36 ). It follows that, conservatively, about half of the microparticles present in the clay fraction of soils in our two study areas have demonstrated capability to adsorb prions and enhance their infectivity [19] , [20] , [26] , and thus could contribute to enhancing the odds of prion infection among deer. Given the wide range of surface area, ionic charge, layer type and expandability among the 'clay minerals' already shown to enhance prion infectivity, it seems plausible that the vast majority of microparticles comprising the clay fraction of soils in our study areas could have some role in prion transmission. Differences in the estimated magnitude of clay's influence on prion infection odds between our two study areas ( Table 1 , Supplementary Tables S1−S2 ) may reflect differences in organic matter or other soil factors, the extent of environmental contamination between areas, differences in seasonal deer mobility and migratory behaviours, or some combination of these (and perhaps other) factors. Despite the plausibility, attempts to link specific soil characteristics to patterns of prion disease occurrence at a broad geographical scale have thus far yielded equivocal results [16] , [17] . Trace elements in soils did not appear to explain observed patterns of scrapie occurrence in the United Kingdom [17] , but soil clay mineralogy data were not considered in that analysis. Analysis of various geochemical factors and their respective influences on scrapie and bovine spongiform encephalopathy incidences in Britain yielded relatively weak evidence of soil clay and organic carbon contents increasing or decreasing, respectively, disease incidence [16] . However, the uniformly low-soil clay content (<5.2%) and low ratio of clay to organic carbon (<2:1) in the soil data analysed, the small sample sizes, and the coarse geographical scale [16] may have precluded or obscured demonstrable effects. Moreover, the common practice of adding phyllosilicate microparticles to livestock feeds [26] could overshadow or confound the influences of soil-derived microparticles on prion transmission risk in production setting as compared with natural systems. Animal traits including genetics, gender, age and mobility all have been shown to influence patterns of prion infection in one or more natural host species [6] , [28] , [29] , [30] , [41] , [42] , [43] . By comparison, the role of environmental factors in prion epidemic dynamics and their potential influence on control strategies are less clear. Shepherds and others familiar with scrapie and its control recognized long ago that environmental factors seemed to influence the perpetuation and recurrence of epidemics [1] , [2] , [3] , [4] . Although scrapie [3] and chronic wasting disease [12] were readily demonstrated to be transmissible from environmental sources, understanding the precise mechanisms and modifiers of environmental transmission of prions has advanced more slowly. For both diseases, observed epidemiological phenomena [3] , [4] , [5] , [6] , [7] , [8] , [9] , [10] , [11] , [12] , [30] , including indirect transmission, persistent infectivity in paddocks and pastures, and interspecies transmission seem best explained by environmental harbouring of prions. Further clarifying whether and how soil and other environmental factors influence prion transmission should complement insights into other aspects of prion biology. The capacity of clay minerals and clay-laden soils to capture and enhance infectivity of shed or deposited prions [19] , [20] , [25] , [26] , [27] and the common tendency of ruminants to ingest soil both deliberately and incidentally in the course of foraging and grooming [12] , [44] , [45] provide an elegantly simple hypothetical mechanism for indirect prion transmission, as follows: infected individuals propagate infectious prions in mucosa-associated lymphoid tissues and shed prions into ingesta and saliva; ingested and environmental soil microparticles with a high phyllosilicate (especially smectite) content bind to, sequester and enhance infectivity of prions both before and after leaving the host; microparticle-bound prions are incorporated into surface soil; susceptible individuals consume contaminated soil and some become infected. (Also see Supplementary Figure S1 .) This mechanism may underlie the apparent importance of indirect transmission in explaining observed patterns of prion infection among captive mule deer [10] , [11] , and perhaps among sheep [3] , [4] , [6] , [7] . In light of these and others' findings, soil clay content and related environmental properties deserve greater attention in assessing local and regional risks of prion disease outbreaks and prospects for their control in natural and production settings. Overview of analytical approach Our study compared the fits of explanatory models to field data from free-ranging mule deer to examine whether soil clay content influenced the odds of an individual deer being prion infected. The hypothesized influence of soil clay was tested while also considering other demographic and habitat factors already known to influence odds of infection in deer [28] , [29] , [30] , [43] . For our analysis, we examined prion infection patterns in mule deer from populations in northern Colorado, United States ( Fig. 2 ). Data were collected from mule deer herds in two geographically separated areas ( Figs 1 and 2 ) in which sample sizes and soil and habitat data were sufficient for analysis. We regarded these study areas as representative of the variation in deer migratory behaviour, disease prevalence and the likely timing of disease introduction seen in other parts of Colorado, as well as elsewhere in western North America where chronic wasting disease is endemic. To estimate the values of habitat variables, we first laid a grid of 3×3 km cells over each study area. For each grid cell, we estimated the average percent of clay-sized (that is, <2 μm) particles in the soil ('percent clay'; Fig. 1 ), the proportion of private land and winter concentration areas, and the distance to nearest riparian habitat. We then overlaid the deer locations reported by hunters onto the landscape grid ( Fig. 1 ). Assuming each deer was killed in its home range and that each 9 km 2 grid cell approximated the size of an average mule deer home range [28] , [29] , we assigned individual deer the habitat covariate values from the respective grid cells where they were killed. To test our original hypothesis that soil clay content would influence the odds of prion infection, we constructed 16 logistic regression models with strictly additive effects ( Supplementary Table S3 ) to represent all possible combinations of demographic, soil clay and other select landscape variables, as well as inherent regional and local spatial structure of the data [29] . All 16 candidate models included age and sex effects because of their well-established influence on infection odds [29] , [30] , [43] . Viewing these 16 models as competing hypotheses, we used the deviance information criterion [29] , [31] , [32] to compare the models' respective fits to the data from sampled deer, and then estimated parameters and examined goodness-of-fit and other metrics for the top model from each data set. We used parameter estimates from the top model for each study area to calculate odds ratios for the effect of soil clay on prion infection odds among deer in that area. A more detailed description of our approach follows. Data sources The Colorado Division of Wildlife provided georeferenced data collected between 2004 and 2008. Each sampled deer was classified by sex, age (<2 years and ≥2 years) and disease status (test-positive or -negative) based on detection of protease-resistant prion protein in lymphoid tissue [46] . The sample for the 7,759 km 2 northcentral study area ( Fig. 1a ) included 2,335 mule deer (202 test-positive, 2,133 test-negative) from six Game Management Units (GMUs) [47] . The sample for the biologically and geographically independent 17,960 km 2 northwestern study area ( Fig. 1b ) included 6,807 mule deer (78 test-positive, 6,729 test-negative) from 16 GMUs. Because we hypothesized a priori that prion infection patterns were structured in part by spatial heterogeneities in features of the landscape, we identified four landscape-level predictors of infection: proportion of clay content in the soil, proportion of private land [29] and winter concentration areas [28] , [29] , and distance to the nearest riparian habitat [29] . To link the disease status (positive or negative) of each deer in the sample to the landscape-level predictors, we first overlaid a square grid having a resolution of 9 km 2 , which is approximately equal to the average home range size for a mule deer in one of our study areas [28] , with the locations of all deer in our study. Previous work had also shown that this movement scale corresponds best to the spatial distribution of prion infection in northcentral Colorado mule deer [29] . There were a total of 862 and 1,995 cells covering the northcentral and northwestern study areas, respectively. We assigned the value associated with each of the four landscape-level predictor variables to deer in our study based on the grid cell that an individual deer was sampled from; thus, all deer sampled from within a particular grid cell were assigned the same value for each landscape-level predictor. The first three landscape predictors were calculated as the cell-level mean proportion of clay content in the soil, proportion of private land and proportion of winter concentration areas. The final landscape variable was calculated as the distance from each grid cell's centre to the nearest riparian habitat. Each of these variables corresponds to our overall a priori hypotheses regarding landscape-level determinants of prion infection within individual mule deer across our study area [29] , [30] , [43] . Therefore, we wanted to specifically investigate the effect of soil clay content on the odds of prion infection adjusted for other covariates already known to have a role in prion epidemic dynamics in deer. We delineated private land using a 1:24,000 map scale of land ownership (for example, federal and private) compiled by the Bureau of Land Management Colorado State Office, and delineated locations of deer wintering concentration areas using information provided by the Colorado Division of Wildlife. Using these spatial data sources, we estimated the proportion (value 0 to 1) of these two covariates in each grid cell using standard Geographic Information Systems (GIS) functions. We measured distance to perennial streams using a 1:24,000 scale hydrological map obtained from the US Geological Survey's Digital Land Graphics. We excluded intermittent streams from our analysis because habitat around streams that held water a majority of the year was likely more influential to deer distribution and prion transmission. We calculated the distance in metres from perennial streams to the centroid of the nearest cell in our 9 km 2 grid. The primary predictor of interest, percent clay (where 'clay' was defined as soil particles with size <2 μm) (ref. 35 ), was determined using the Advanced Mode of the Soil Data Viewer in ArcMap available through the National Resources Conservation Service of the US Department of Agriculture [37] . Soil Data Viewer provides interactive mapping software to query the Soil Survey Geographic (SSURGO) database and descriptive characteristics for each soil type [35] , [48] . Clay was expressed as the percent clay within a soil type polygon ( ∼ 2 ha resolution) for each soil map unit [35] , [48] . Because each grid cell was typically composed of multiple soil type polygons, with each soil type having its own estimated clay content, we used a weighted average based on the proportion of the total area occupied by each unique soil type within a grid cell to estimate the mean proportion of soil clay content in each 9 km 2 cell. Statistical analysis. We analysed data from the northcentral Colorado GMUs independently from the data from northwestern Colorado GMUs, because of their geographical separation and differences in deer migratory behaviour, prion disease prevalence and the likely timing of prion disease introduction into each region. We used a Bayesian hierarchical model structure [51] , [52] to examine how soil clay content influenced the probability of an individual deer being infected, while adjusting for the other covariates and spatial structure in the data [29] . To adjust for latent spatial effects we included two types of random effects that captured both the influence of the local neighbourhood (that is, cells sharing a border or vertex with each 9-km 2 grid cell) in determining spatial clustering of CWD, as well as any spatially independent influences occurring at the 9 km 2 spatial resolution of our grid representing an individual deer home range [29] , [49] , [50] . Our models were constructed hierarchically to accommodate the fact that information from multiple levels (that is, fixed-effects and spatial random effects) was being used to estimate individual-level infection probabilities. Taking a Bayesian approach, we used Markov Chain Monte Carlo simulation methods available within the programme WinBUGS [53] to produce the unnormalized joint posterior density for the parameters of interest across all models examined based on the product of the data likelihood and the prior densities for each parameter. We used this approach to estimate the posterior marginal probability distributions for the parameters governing the influence of the demographic, landscape-level and spatial random effects predictors on the probability of infection. For each model we ran three independent Markov chains with varying initial values for 350,000 iterations and discarded the first 100,000. We thinned the Markov chains by keeping every twentieth iteration for inference. To determine whether the three Markov chains used for each model had converged on the same posterior distribution, we used the statistical programme R [54] with the package boa [55] and used several graphical and quantitative diagnostics, including autocorrelation plots, trace plots and univariate corrected scale reduction factors for each parameter. To assess simultaneous convergence of all parameters for the top models, we calculated the multivariate potential scale reduction factor [52] , [56] , [57] . All inferences were based on the mean of each parameter's marginal posterior distribution. Details of our likelihood functions [51] and prior distributions [51] , [52] , [58] , [59] , [60] are provided as Supplementary Methods . How to cite this article: Walter, W. D. et al . Soil clay content underlies prion infection odds. Nat. Commun. 2:200 doi: 10.1038/ncomms1203 (2011).